Local orthogonality as a multipartite principle for quantum correlations In recent years, the use of information principles to understand quantum correlations has been very successful. Unfortunately, all principles considered so far have a bipartite formulation, but intrinsically multipartite principles, yet to be discovered, are necessary for reproducing quantum correlations. Here we introduce local orthogonality, an intrinsically multipartite principle stating that events involving different outcomes of the same local measurement must be exclusive or orthogonal. We prove that it is equivalent to no-signalling in the bipartite scenario but more restrictive for more than two parties. By exploiting this non-equivalence, it is then demonstrated that some bipartite supra-quantum correlations do violate the local orthogonality when distributed among several parties. Finally, we show how its multipartite character allows revealing the non-quantumness of correlations for which any bipartite principle fails. We believe that local orthogonality is a crucial ingredient for understanding no-signalling and quantum correlations. Understanding the structure of correlations within our current description of nature, based on quantum physics, is a fundamental open problem. In particular, one would like to characterize the set of quantum correlations, that is, correlations which can result from local measurements on quantum states. Pioneering work by Popescu and Rohrlich [1] showed that the no-signalling (NS) principle—that is, the impossibility of instantaneous communication—does not suffice to recover this quantum set. Indeed, they provided examples of correlations between two parties compatible with the NS principle but without any quantum realization. The most paradigmatic example of these supra-quantum correlations is the so-called Popescu-Rohrlich (PR) box, also studied by Tsirelson [2] . The search for better principles separating supra-quantum correlations from quantum ones, or ideally a complete characterization of the quantum set, was started. An important boost to this search was because of Van Dam [3] , who introduced the idea that the existence of supra-quantum correlations, while not violating the NS principle, could have implausible consequences from an information-processing point of view. Van Dam [3] showed that distant parties having access to PR-boxes can render communication complexity trivial and argued that this could be a reason for the non-existence of these correlations in nature. Since then, intensive effort has been devoted to the search for information principles characterizing the set of quantum correlations, for example, the aforementioned non-trivial communication complexity [3] , [4] , information causality [5] and macroscopic locality [6] . Recently, it has been shown that intrinsically multipartite principles are essential to characterize the set of quantum correlations. It was proven by Gallego et al. [7] that there exist supra-quantum correlations for three parties that cannot be detected by any bipartite principle. Unfortunately, most of the existing principles for quantum correlations are formulated in a bipartite setting and their multipartite generalization is unclear, apart from the trivial one in which the parties are split in two groups and the principle is applied to each bipartition. In this sense, note that even the NS principle has a bipartite formulation in the multipartite scenario: correlations among n distant parties satisfy the NS principle whenever the marginal distribution seen by a subset of the n parties is independent of the choice of measurements by the remaining ones. In this work, we introduce the concept of local orthogonality (LO), an intrinsically multipartite principle for correlations. The principle is based on a definition of orthogonality (or exclusiveness) between events involving measurement choices and results by n distant parties: we define some events to be orthogonal, or exclusive, whenever they involve different outcomes of the same local measurement by at least one of the parties. Operationally, we demand that the sum of the probabilities of mutually exclusive events is less than or equal to one, which implies a restriction on possible correlations. We provide an information-processing interpretation of this new principle in terms of a distributed guessing problem (DGP). We then show how the principle implies a highly non-trivial structure in the space of correlations. First, we prove that, whereas the set of LO correlations coincides with the set of NS correlations for two parties, it is strictly smaller for more than two parties. Second, by exploiting the non-equivalence of LO and the NS principle in the multipartite case, it is demonstrated how LO can also be used to detect the non-quantumness of some supra-quantum, bipartite NS correlations. In particular, we prove that distributed copies of the PR-box violate LO, and show how one can get very close to the boundary of the quantum set of bipartite correlations (Tsirelson's bound) by imposing LO. Finally, we prove that the intrinsically multipartite formulation of the principle allows one to detect supra-quantum correlations for which any bipartite principle fails. In deriving all these results, we exploited a connection between LO correlations and graph theory, related to the constructions derived by Cabello et al. [8] in the study of quantum contextuality. In fact, there is a natural notion of orthogonality (also called ‘exclusiveness’) between events in contextuality scenarios, which are defined by sets of measurements sharing some measurement outcomes (two events are orthogonal if they correspond to different outcomes of a given measurement). For instance, several works have studied how the violation of the corresponding orthogonality conditions can lead to supra-quantum correlations [9] , [10] , or how these orthogonality conditions can be used to provide upper bounds to the quantum violation of non-contextuality inequalities [8] . Definition We start by presenting the formal definition of the LO principle in a general Bell scenario involving n distant parties, each of them having an access to a physical system. Each party can perform m different measurements on the system, getting one out of d possible outcomes. This scenario is denoted by ( n , m , d ). The measurement applied by party i is denoted by x i , and the corresponding outcome by a i , with i ∈ {1, …, n }, x i ∈ {0, …, m −1} and a i ∈ {0, …, d −1}. The correlations among the parties are described by the joint conditional probability distribution P ( a 1 … a n | x 1 … x n ), representing the probability for the parties to get outcomes a 1 , …, a n when making measurements x 1 , …, x n . The main aim of LO is to introduce a notion of exclusiveness in the space of events. Consider first two different events e and e ′ given by e =( a 1 … a n | x 1 … x n ) and e ′=( a 1 ′… a n ′| x ′ 1 … x ′ n ). We call these two events locally orthogonal or simply orthogonal, if they involve different outputs of the same measurement by (at least) one party; that is, if for some i we have a i ≠ a i ′ whereas x i = x i ′. We then call a collection of events { e i } orthogonal, or exclusive, if the events are pairwise orthogonal, and impose that for any set of orthogonal events, the sum of their probabilities must not be larger than one, This requirement is the LO principle. To summarize: the LO principle (i) introduces a notion of orthogonality between two events, (ii) imposes that any number of events are orthogonal whenever they are pairwise orthogonal and (iii) requires that the inequality (1) is satisfied for any set of orthogonal events. The notion of orthogonality is rather natural in the case of two events, and the requirement (1) is automatically satisfied for NS correlations. In fact, consider two LO events e 1 , e 2 with a i ≠ a i ′ and x i = x i ′ as before. These two events can be seen as different outcomes of a correlated measurement in which: (i) party i first measures x i and announces the outcome to the other parties and (ii) the other parties apply measurements depending on this outcome, in particular they measure x 1 , …, x n , if the outcome is a i , and x ′ 1 , …, x ′ n otherwise. Thus, as e 1 and e 2 are outcomes of the same (correlated) measurement, the requirement (1) immediately follows from normalization. Note that the NS principle is essential for this correlated measurement to be meaningful, as it is possible to define the marginal probability for party i in the first step of the correlated measurement independently of the successive actions by the other parties. The principle, however, becomes more restrictive when considering more events, in which the previous reasoning does not apply any longer. As mentioned above, we extend the initial definition of orthogonality for two events to more events by demanding pairwise orthogonality. It is precisely this extended and intrinsically multipartite formulation that makes the principle non-trivial, as it involves summing probabilities conditioned on different measurements. Taken together, all the restrictions on the conditional probability distributions implied by LO define the set of LO inequalities (1) for the ( n , m , d ) scenario. The set of LO correlations is then the set of conditional distributions P ( a 1 … a n | x 1 … x n ) satisfying all the LO inequalities. Moreover, we can define the sets of conditional probability distributions that obey LO for a certain number of copies in the following sense. A given distribution for the ( n , m , d ) scenario can be thought of as provided by some device shared between the n parties, each having access to one input and output of the device. If the distribution provided by the device is compatible with LO, a natural question is whether a larger distribution coming from several copies of such a device distributed among more parties necessarily satisfies LO. As we will explain below, the answer to this question is negative; that is, LO displays activation effects and, hence, we have a hierarchy of sets. The largest set in this hierarchy, denoted , is the set of all distributions in the ( n , m , d ) scenario that obey the LO inequalities for this scenario. Now consider k copies of a device characterized by a distribution P , distributed among kn parties, each of which has access to one input of only one device. If the distribution P k of the kn -partite global device obeys all the LO inequalities for the scenario ( kn , m , d ), we say that P satisfies LO k , and belongs to . We denote by the set of distributions for ( n , m , d ) that obey the LO inequalities for any number of copies. Having stated the LO principle, our main goal is the study of the sets of LO correlations. As we shall see, the LO principle turns out to be very powerful for ruling out non-quantum correlations. As in the case of contextuality [8] , graph theory is perfectly suited for our purposes. We consider the ( md ) n possible events in the ( n , m , d ) scenario and map them on an orthogonality graph with ( md ) n vertices, where two vertices are connected by an edge if and only if the corresponding events are locally orthogonal. For instance, Fig. 1 shows the orthogonality graph of the (2, 2, 2) scenario. In the graph theory, a clique in a graph G =( V , E ) is a subset of vertices C ⊆ V such that the subgraph induced by C is complete, that is, such that all pairs of vertices in C are connected by an edge in G . A clique is maximal if it cannot be extended to another clique by including a new vertex. Clearly, any clique in the orthogonality graph of events gives rise to an LO inequality (and vice versa), as all events in the clique are connected and, thus, are pairwise orthogonal. Therefore, the problem ‘find all the optimal LO inequalities’ is equivalent to ‘find all maximal cliques of the associated orthogonality graph’. While the problem of finding all maximal cliques of a graph is known to be NP-hard [11] , there exist software packages [12] , [13] that provide the solution for small graphs. We have used these packages to derive and partly classify LO inequalities for various Bell scenarios, which will be presented elsewhere. Note, however, that in principle, while the problem of finding the maximal cliques is NP-hard for general graphs, this may no longer be the case for graphs associated to correlations among distant parties. Indeed, these graphs may represent a subset of all possible graphs that does not include the hard instances of the problem. 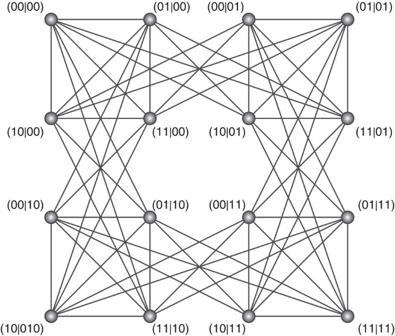Figure 1: Orthogonality graph of the (2,2,2) scenario. As mentioned in the text, each possible event corresponds to a node, whereas the edges connect locally orthogonal events. Figure 1: Orthogonality graph of the (2,2,2) scenario. As mentioned in the text, each possible event corresponds to a node, whereas the edges connect locally orthogonal events. Full size image Distributed guessing problems Before moving on to the characterization of LO correlations, we provide an interpretation of the principle from an information-processing viewpoint. To this end, we introduce the notion of a DGP. Guessing problems are ubiquitous in science. In the standard formulation (see Fig. 2a ), an observer has the access to some data x , which depends on some initial parameter ã , that is x = f ( ã ). From the observed data, the observer should make a guess, a , of the initial parameter. His goal is to maximize the probability of guessing correctly. 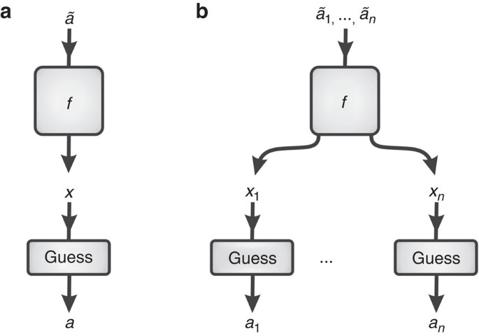Figure 2: Distributed guessing problems. In the standard scenario (a), an observer has to guess the value of a parameterãgiven only some function of it,x=f(ã). In the distributed scenario (b), the input parameter is a vector ofnsymbols, (ã1, ,ãn), and so are the data given to the players (x1, …,xn). Each of player has an access to just one of the symbolsxjand has to guess the corresponding initial parameterãj. The game is won when all the players guess correctly. Figure 2: Distributed guessing problems. In the standard scenario ( a ), an observer has to guess the value of a parameter ã given only some function of it, x = f ( ã ). In the distributed scenario ( b ), the input parameter is a vector of n symbols, ( ã 1 , , ã n ), and so are the data given to the players ( x 1 , …, x n ). Each of player has an access to just one of the symbols x j and has to guess the corresponding initial parameter ã j . The game is won when all the players guess correctly. Full size image Guessing problems can be easily adapted to distributed scenarios. It is convenient to present the DGP as a game and to phrase it in terms of vectors of symbols. Consider then a non-local game in which a referee has access to a set of vectors of n symbols with values in {0, …, d −1}. Denote this set by S and its size by | S |, which can be less than d n in general. Now, the referee chooses a vector ( ã 1 , …, ã n ) uniformly at random from S , and encodes it into a new vector of, again, n symbols using a function f . However, the new symbols can now take m values and, thus, f : S → {0, …, m− 1} n . The resulting vector is ( x 1 , …, x n )= f ( ã 1 , …, ã n ). These n symbols are distributed among n distant players who cannot communicate and must produce individual guesses a 1 , …, a n . Their goal is to guess the initial input to the function, that is, they win whenever a j = ã j for all j . Note that the encoding function f and the set S are known in advance to all the players. For some f , for example, for x j = ã j , this task is very simple. However, there exist functions for which the task becomes extremely difficult. For a fixed size | S |, the most difficult functions are those for which the maximum guessing probability is equal to 1/| S |. The players can always achieve this guessing probability by agreeing beforehand on one of the | S | possible outputs, regardless of the x j . As the input is uniform on S , their guess is correct with probability 1/| S |. A DGP is thus maximally difficult whenever this strategy is optimal, that is, whenever it is impossible to provide a better estimate of the input than random guessing. For such an f , having access to the symbols x j does not provide any useful information to the parties. Note that non-trivial maximally difficult functions are possible only in distributed scenarios. In standard single-observer guessing problems, the only maximally difficult function is the one defined by a constant function f , which trivially erases any information about the input. An example of a difficult function in the ( n , 2, 2) scenario for odd n and classically correlated players is f ( a 1 , …, a n )=( a n , a 1 , …, a n −1 ) defined on the set S of inputs satisfying a 1 ⊕ … ⊕ a n =0. This is the guess-your-neighbour’s-input task considered in the work by Almeida et al. [14] As we prove in Methods, a DGP is maximally difficult for players sharing classical correlations (classical players) if, and only if, it corresponds to an LO inequality. Hence, in order to win the game with a probability larger than 1/| S |, they need to share correlations violating LO. In particular, quantum correlations provide no advantage over the trivial strategy of randomly guessing the solution. The NS principle The first question we ask while characterizing LO correlations is how they relate to the set of NS correlations, denoted by . For bipartite scenarios, the two principles define the same set of correlations, as was already noticed in the work of Cabello et al. [8] (in Methods, we give a slightly different proof that emphasizes the connection with LO). However, the equivalence between LO and NS breaks down while moving to the multipartite scenario. We exploited the graph-theoretical approach mentioned in the previous section to generate the list of LO inequalities for different scenarios, and then classified them into equivalence classes under relabellings, permutations of parties and NS constraints (using a Mathematica as well as MATLAB code kindly provided to us by J.D. Bancal). Already in the simplest tripartite scenario (3, 2, 2), we find one and only one class of non-trivial LO inequalities, in which non-trivial means that the inequalities are violated by some NS correlations. This inequality turns out to be the GYNI inequality [14] , which in the tripartite case reads P (000|000)+ P (110|011)+ P (011|101)+ P (101|110)≤1. It is easy to see by simple inspection that GYNI is an LO inequality. As shown in the studies of Almeida et al. [14] , the maximum of the GYNI inequality over is equal to 4/3. Our numerical data suggest that the gap between and increases with the number of parties: in the (4, 2, 2) scenario, we find 35 equivalence classes. Unfortunately, for more parties ( n >4), even the simplest scenario ( n , 2, 2) becomes computationally intractable because of the large size of the orthogonality graph. Nevertheless, examples of such inequalities for larger n as well as m and d are known and can be constructed from unextendible product bases [15] by using the method discussed in Augusiak et al. [16] , [17] (see also the work of Acin et al. [18] ). It is worth mentioning that all the known examples of non-trivial, tight (in the sense of defining a tight Bell inequality [19] ) information tasks with no quantum advantage, given in Almeida et al. [14] , Augusiak et al. [16] , [17] , Acín et al. [18] , are examples of LO inequalities. It is an interesting working conjecture to prove that any non-trivial and tight information task with no quantum advantage defines an LO inequality. In particular, this would imply that any non-trivial tight Bell inequality in a bipartite scenario has quantum violations. Supra-quantum correlations The LO principle is naturally satisfied by quantum correlations. Indeed, orthogonal events can be associated with measurements described by projectors with disjoint supports (see Methods for details). We now investigate the use of the LO principle as a tool to detect post-quantum NS correlations. Clearly, those correlations violating GYNI are in contradiction with LO as well. However, the situation turns out to be much richer, already for two parties. In principle, one might think that LO would be useless for the detection of supra-quantum bipartite correlations because of the equivalence with NS. However, this intuition is not correct. We can show that postulating LO also on the many-party level leads to the detection of non-quantumness of bipartite correlations. Given some bipartite correlations, the main idea consists of distributing k copies of these among 2 k parties, such that one party has access to one part (input and output) of only one bipartite box. In the resulting 2 k -partite scenario, the LO principle is stronger than the NS principle. Thus, it may happen that the initial bipartite correlations violate LO when distributed among different parties in a network. The idea is similar in spirit to the network approach to non-locality presented by Cavalcanti et al. [20] A PR-box is a hypothetical device taking binary inputs and giving binary outputs, which obey PR ( ab | xy )=1/2 if a ⊕ b = xy and PR ( ab | xy )=0 otherwise [1] . These boxes are known to be more non-local than what quantum theory allows. For instance, they provide a violation of the Clauser–Horne–Shimony–Holt Bell inequality [21] larger than Tsirelson's bound for quantum correlations [22] . PR-boxes are bipartite NS devices, and therefore might naively be expected to satisfy LO. However, we prove now that when distributed in networks they violate LO. Consider k copies of a PR-box, distributed among 2 k parties as shown in Fig. 3 . 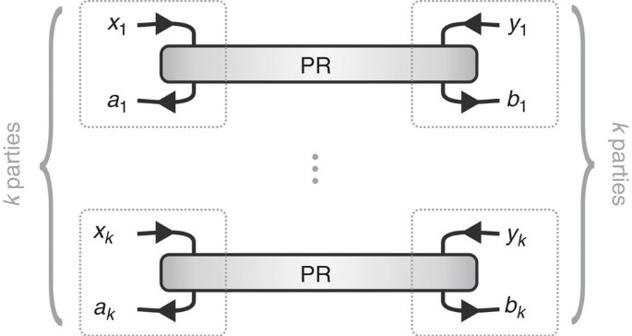Figure 3: Network of PR-boxes. We considerkcopies of a PR-box shared among 2kparties. Each party has an access to one part of a box. The conditional probability distribution is: Figure 3: Network of PR-boxes. We consider k copies of a PR-box shared among 2 k parties. Each party has an access to one part of a box. Full size image where j labels the k boxes. Already for k =2, we find LO inequalities violated by these two copies of the PR-box, and hence PR-boxes do not satisfy LO 2 . One example of such an inequality is P (0000|0000)+ P (1110|0011)+ P (0011|0110)+ P (1101|1011)+ P (0111|1101) ≤1. For a PR-box, the left-hand side is equal to 5/4. We can also analyse noisy versions of the PR-box given by P q = qPR +(1− q ) , where ( ab | xy =1/4) for all a , b , x , y . We find that two copies of a noisy PR-box violate LO down to q ≈0.72, which is close to Tsirelson's bound (meaning that noisy boxes with can be simulated with quantum states and measurements). Detailed derivations of these results are presented in Methods. An immediate consequence of these results is that LO also rules out all extremal boxes in the (2, 2, d ) and (2, m , 2) scenarios. The first case follows from the fact that any extremal box in the (2, 2, d ) case can always be used to simulate a PR-box arbitrarily well [23] . For the (2, m , 2) scenario, all the extremal boxes were characterized by Jones et al. [24] (see also the work by Barrett et al. [25] ). There, it is shown that, up to symmetries, an extremal non-local box is equivalent to a PR-box if one restricts the considerations to the first two inputs out of the m possible choices. Hence, any LO inequality violated by a PR-box is also violated by any extremal non-local bipartite binary box. It is also interesting to compare LO with information causality (IC) [5] , another proposal for a physical principle to single out quantum correlations. A natural question then is whether and when LO can do better than IC in ruling out supra-quantum correlations. Following Allcock et al. [26] , we study LO predictions for different families of NS correlations. In some situations, LO provides a bound to the set of quantum correlations which is tighter than the known bounds obtained from applications of IC, as can be seen in Fig. 4 . Hence, LO rules out correlations that were not excluded before by IC. 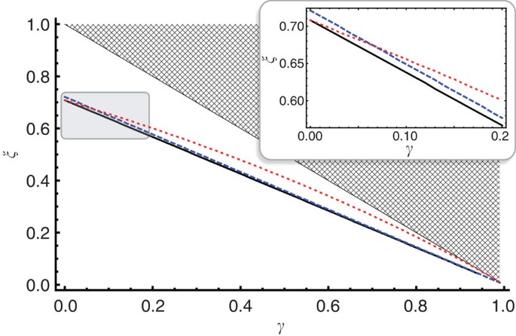Figure 4: IC versus LO performance. Comparison of both principles for detecting supra-quantum correlations in the (2,2,2) scenario. We consider the family of correlations parametrized as, wherePL(ab|xy)=δa,0δb,0. The curves show the bounds provided by the 1+AB level of the NPA hierarchy32,33(black), LO2(blue dashed), IC (red dotted) and the edge of the crossed-out region corresponds to NS correlations and bounds that allowed parameter space. Note that when γ→0 (see inset), IC approximates the quantum set better than LO2, which is consistent with the fact that IC recovers Tsirelson’s bound for γ=0, whereas LO reaches ≈0.72 for two copies of the device. However, LO beats the known IC bound for other parameter values, ruling out correlations that were not excluded before. Figure 4: IC versus LO performance. Comparison of both principles for detecting supra-quantum correlations in the (2,2,2) scenario. We consider the family of correlations parametrized as , where P L ( ab | xy )=δ a ,0 δ b ,0 . The curves show the bounds provided by the 1+AB level of the NPA hierarchy [32] , [33] (black), LO 2 (blue dashed), IC (red dotted) and the edge of the crossed-out region corresponds to NS correlations and bounds that allowed parameter space. Note that when γ→0 (see inset), IC approximates the quantum set better than LO 2 , which is consistent with the fact that IC recovers Tsirelson’s bound for γ=0, whereas LO reaches ≈0.72 for two copies of the device. However, LO beats the known IC bound for other parameter values, ruling out correlations that were not excluded before. Full size image So far, we have focused on how some bipartite supra-quantum correlations can be excluded by LO. Owing to the intrinsically multipartite formulation of the principle, we expect it to be of particular relevance for the study of genuine multipartite correlations among more than two parties. As an example, we study how well LO performs for extremal NS non-local correlations in the (3, 2, 2) scenario. All these extremal NS boxes were computed by Pironio et al. [27] and any NS correlations in this scenario can be obtained by mixing them. These extremal boxes can be grouped into 46 equivalence classes under symmetries, the first class corresponding to deterministic local points, whereas the other 45 are non-local. The latter can be interpreted as the maximally non-local correlations in the (3, 2, 2) scenario compatible with the NS principle. LO can be shown to rule out all these maximally non-local boxes. We follow a method similar to the one for PR-boxes presented in Methods, although for some cases the tripartite boxes required a slightly more general approach in terms of weighted graphs. The details of these derivations are beyond the scope of the present manuscript and will be presented elsewhere. We find that every maximally non-local box in (3, 2, 2) violates either LO 1 or LO 2 , and hence cannot have a quantum realization. We conclude this part with a couple of observations. First, LO is, to our knowledge, the first principle able to rule out all the known examples of extremal non-local boxes. We have shown it first for the only maximally non-local box in the (2, 2, 2) scenario (the PR-box), then for maximally non-local boxes in the (2, m , 2) and (2, 2, d ) scenarios, as well as for all extremal boxes in the (3, 2, 2) case. Second, the intrinsically multipartite formulation of LO allows detecting correlations, for which any bipartite principle fails. For instance, the correlations provided by Gallego et al. [7] violate GYNI and, consequently, also LO, but satisfy every bipartite principle. Moreover, box number 4 described in Pironio et al. [27] is an example of a tripartite NS box, which cannot be ruled out by any bipartite principle [28] , but which violates LO. Multipartite principles are necessary to understand the structure of quantum correlations from an information perspective. Local orthogonality is a principle for correlations that has an intrinsically multipartite formulation. It has a natural interpretation in terms of DGPs. Moreover, it can be used in the study of correlations by applying standard techniques from graph theory. We have shown here that the principle gets very close to the set of quantum correlations and detects all known maximally non-local boxes as supra-quantum, including those for which any bipartite principle fails. We believe that LO will be an essential ingredient for the characterization and understanding of correlations. An intriguing question is to understand the exact relation between this set and the set of quantum correlations. Miguel Navascués first noticed that the set of quantum correlations is strictly smaller than , as also proved by Fritz et al. [29] Are there simple additional principles that, together with LO, completely characterize the set of quantum correlations? Another interesting line of research consists in extending our approach, here formulated for Bell scenarios, to other frameworks. In fact, the principle is rather general: after introducing a notion of orthogonality in a space of events, the whole machinery of graph theory and copies of the graph (networks) automatically applies. A natural framework for its application is the study of contextuality scenarios where, as mentioned, there is a natural notion of orthogonality (or exclusiveness). In fact, our approach has successfully been applied to the study of quantum contextuality in several recent works [29] , [30] , [31] . Maximally difficult DGPs and LO inequalities Our goal here is to prove that imposing that correlations do not provide any advantage for DGP involving maximally difficult functions f is equivalent to LO. For such an f and any correlations P ( a 1 … a n | x 1 … x n ), providing no advantage for the DGP defined by f means that where f 1 , …, f n refer to the components of the vector f , and x j = f j ( a 1 , …, a n ) is the input that party j receives. Note that, for simplicity, and as the goal of the parties is to provide a correct guess of the initial parameters, we slightly abuse notation and replace all ã j by a j . In order to prove the correspondence, we now show that functions f that are maximally difficult for classical players are precisely those which have the property that if f ( a 1 , …, a n ) and f ( a ′ 1 , …, a ′ n ) are both defined, then there exists some j for which a j ≠ a ′ j , but f j ( a 1 , …, a n )= f j ( a ′ 1 , …, a ′ n ). Given that f varies over all those partial functions having this property, the DGP inequalities (3) define all LO inequalities in the ( n , m , d ) scenario. We first prove the ‘only if’ direction by contradiction. Assume there exist a 1 , …, a n and a ′ 1 , …, a ′ n , in both of which f is defined such that for every party j either a j = a ′ j or f j ( a 1 , …, a n )≠ f j ( a ′ 1 , …, a ′ n ) holds true. Then the following classical strategy performs better than random guessing: for those j with a j = a ′ j , let them output this particular value independently of their input; for those with a j ≠ a ′ j and f j ( a 1 , …, a n )≠ f j ( a ′ 1 , …, a ′ n ), choose some function g j such that a j = g j ( f j ( a 1 , …, a n )) and a ′ j = g j ( f j ( a ′ 1 , …, a ′ n )), and let them output g j ( x j ). This strategy recovers all correct values both for the a 1 , …, a n as well as for the a ′ 1 , …, a ′ n , and therefore performs better than random guessing. Conversely, we need to show that if f has this property, then using local operations only cannot be more successful than random guessing. Thanks to convexity, it is enough to consider deterministic local strategies. If a deterministic strategy is better than random guessing, there needs to exist at least a 1 , …, a n and a ′ 1 , …, a ′ n such that the strategy works on both of these. In particular, this means that, for each party j , either a j = a ′ j , or party j needs to be able to tell the two cases apart via x j , so that f j ( a 1 , …, a n )≠ f j ( a ′ 1 , …, a n ). This implies that f cannot have the property described above. NS and LO 1 in bipartite scenarios We prove that in the bipartite case, LO 1 and NS define the same set of correlations. Although this is already known [8] , here we give a slightly different proof that emphasizes the connection with LO. To simplify the notation, in the bipartite scenario, measurements and results by the two parties are labelled by x , y and a , b , so that correlations read P ( ab | xy ). Let us start by characterizing the possible sets of locally orthogonal events. Recall that two events are locally orthogonal if for at least one party the settings are identical but the outcomes are different. Consider a set of locally orthogonal events that contains ( ab | xy ) and ( a ′ b ′| x ′ y ) with x ′≠ x . Then, this set cannot contain any event of the form ( a ′′ b ′′| x ′′ y ′) with y ′≠ y , as it could not be locally orthogonal to both other events. From this intuition, we find that the sets of pairwise orthogonal events are either {( ab | xω A ( a )): a , b =0, …, d −1} for fixed x , or {( ab | ω B ( b ) y ): a , b =0, …, d −1} for fixed y with ω W : {0, …, d −1}→{0, …, m −1} ( W = A , B ) being some map. We start by showing that sets of the first kind have the desired property; the proof for sets of the second kind is analogous. Take two such events ( ab | xω A ( a ))≠( a ′ b ′| xω A ( a ′)). Then, either a ≠ a ′ and orthogonality holds on Alice’s side, or b ≠ b ′ and orthogonality follows from Bob. This proves that we have a set of LO events. To see that the set is maximal, consider an arbitrary event . If and , then this event is already in the set. Otherwise, LO fails between and . Hence, it is impossible to add any event to the set, that is, the set is maximal. Now we prove that every maximal LO 1 set is of one of these two forms. It is enough to show that every LO 1 set is contained in a set of this form. As noted above, for events in an LO set, one of the parties is restricted to using a single input. Hence, without the loss of generality, we can take x to be fixed. As every two orthogonal events differ on at least one outcome, there exists a function ω ( a , b ), such that every element in the set is of the form ( ab | xω ( a , b )). We complete the proof by showing that ω ( a , b ) does not depend on b . The existence of a and b , b ′ with ω ( a , b )≠ ω ( a , b ′) would imply that ( ab | xω ( a , b )) and ( ab ′| xω ( a , b ′)) are not orthogonal, contradicting the assumption. We denote by the set of distributions P ( ab | xy ) satisfying NS. The conditions for NS are and we also have the normalization conditions , ∀ x , y . We now prove that in the present bipartite setting. : all optimal LO 1 inequalities are of the form , modulo exchanging the parties. We fix any a 0 , y and y ′ and consider the function ω A ( a )= y , if a = a 0 and ω A ( a )= y ′ if a ≠ a 0 . The LO inequality yields . Together with the normalization equation , this implies . As the same inequality can be derived with y and y ′ interchanged, we find that it actually needs to be an equality, which is (4). : start from the normalization condition . Using the NS equation (4), we can transform it into an equality of the form for any given x and ω A . It follows that , and thus , in the bipartite scenario. Quantum correlations satisfy LO It is straightforward to see that LO inequalities are satisfied by the set of quantum correlations, denoted , that is, . For simplicity, we give the proof for an inequality involving two LO events. The generalization to an arbitrary LO inequality, and in particular to any number of copies is straightforward and follows from the property that in quantum mechanics, a set of projective measurements that can be pairwise implemented, can be jointly implemented (that is, pairwise orthogonality between projectors implies orthogonality of all the projectors). Consider two LO events e 1 =( a 1 … a n | x 1 … x n ) and e 2 =( a ′ 1 … a ′ n | x ′ 1 … x ′ n ) with a i ≠ a ′ i , x i = x ′ i , and the corresponding inequality p ( e 1 )+ p ( e 2 )≤1. The maximization of the sum of these two probabilities over quantum correlations reads where the maximization runs over all possible states |Ψ〉 and projectors acting on an arbitrary Hilbert space. Note that the maximization can be carried out over projective measurements without the loss of generality, as the ancilla needed for a general measurement can be absorbed in the definition of the state |Ψ〉. The term in the parenthesis is equal to the sum of two orthogonal projectors, as . Thus, this sum is upper bounded by the identity operator and the LO inequality follows. Two PR-boxes violate LO We classify events as either ‘possible’ or ‘not possible’ for this many-copy box as follows. An event ( ab | xy ) for one PR-box is possible if a ⊕ b = xy . Hence, PR-box correlations may be written as In the case of k boxes, an event ( a 1 b 1 ⋯ a k b k | x 1 y 1 ⋯ x k y k ) is possible if a j ⊕ b j = x j y j for all j ∈ {1, …, k }. Then, the general form for the k -box probability (2) is Consider a clique C ⊆ V in the orthogonality graph G =( V , E ) of the scenario (2 k , 2, 2) and the corresponding LO inequality LO ( C ). Define the set C p ⊆ C to be the subset of possible events in C . Then, the multipartite box (7) violates LO ( C ) if, and only if, it violates LO ( C p ). In particular, in order to exclude the PR-box, it is sufficient to find a clique of size larger than 2 k in the orthogonality graph G poss =( V p , E p ) of possible events for box (7). This problem becomes significantly easier, as | V p |=8 k , compared with | V |=16 k , for the initial graph (compare Figs 1 and 5 ). Already for k =2, there exist cliques of size larger that 4. We found that all of them have size 5, and one example is given by: {(0000|0000), (1110|0011), (0011|0110), (1101|1011), (0111|1101)}. 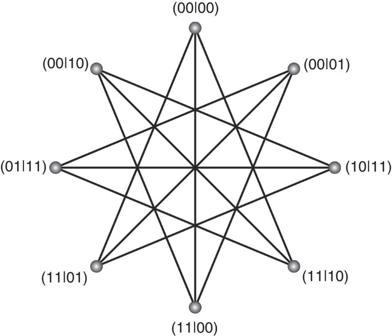Figure 5: Orthogonality graph of possible events for a single PR-box. It coincides withFigure 2in the work of Sadiqet al.34, in which the authors studied the CHSH inequality. Figure 5: Orthogonality graph of possible events for a single PR-box. It coincides with Figure 2 in the work of Sadiq et al. [34] , in which the authors studied the CHSH inequality. Full size image Consider now two copies of a noisy PR-box given by P q = qPR +(1− q ) , where ( a,b | x,y )=1/4 for all a , b , x , y . Now all events become possible and one should consider the full list of LO inequalities for (4, 2, 2). However, one can still consider this five-term inequality as associated to a non-maximal clique in the orthogonality graph of the (4, 2, 2) scenario, and complete it to a maximal clique. This gives an inequality with additional terms corresponding to events that are impossible for the PR-box, but which are possible for a noisy PR-box. In this way, we have found that the distribution violates LO for q ≳ 0.72. An example of such an LO inequality is given by the following set of 10 LO events: {(1111|0000), (1100|1010), (0100|1100),(0011|0001), (0010|0111), (1011|0000), (0101|1100), (1101|1100),(1010|0110), (1001|0100)}. It appears plausible to conjecture that the generalization of the previous approach to an arbitrary number of parties converges to Tsirelson’s bound in the limit of an infinite number of parties, although we did not yet find any proof. How to cite this article: Fritz, T. et al. Local orthogonality as a multipartite principle for quantum correlations. Nat. Commun. 4:2263 doi: 10.1038/ncomms3263 (2013).